A reconfigurable plasmofluidic lens Plasmonics provides an unparalleled method for manipulating light beyond the diffraction limit, making it a promising technology for the development of ultra-small, ultra-fast and power-efficient optical devices. To date, the majority of plasmonic devices are in the solid state and have limited tunability or configurability. Moreover, individual solid-state plasmonic devices lack the ability to deliver multiple functionalities. Here we utilize laser-induced surface bubbles on a metal film to demonstrate, for the first time, a plasmonic lens in a microfluidic environment. Our ‘plasmofluidic lens’ is dynamically tunable and reconfigurable. We record divergence, collimation and focusing of surface plasmon polaritons using this device. The plasmofluidic lens requires no sophisticated nanofabrication and utilizes only a single low-cost diode laser. Our results show that the integration of plasmonics and microfluidics allows for new opportunities in developing complex plasmonic elements with multiple functionalities, high-sensitivity and high-throughput biomedical detection systems, as well as on-chip, all-optical information processing techniques. The field of plasmonics has become a very active branch in nanophotonics [1] , [2] . Utilizing the unique properties of surface plasmon polaritons (SPPs), which occur at the interface of metals and dielectrics [3] , plasmonic devices are capable of confining light in dimensions smaller than the Abbe diffraction limit and implementing extremely large field enhancement. Significant progress has been achieved in the field of plasmonics, ranging from super-resolution imaging [4] , [5] , [6] , [7] , [8] , plasmonic circuits [9] , [10] , [11] and energy harvesting [12] , [13] to ultra-sensitive biochemical detection [14] , [15] and optical metamaterials [16] , [17] . However, until recently, most plasmonic devices were built on metals and dielectrics in solid state and lacked tunability and reconfigurability. Extensive effort has been devoted to active plasmonics in an attempt to dynamically control the resonance or propagation of surface plasmons by various functional media and response mechanisms [18] , [19] , [20] , [21] , [22] . Optofluidics (that is, fusion of optics and microfluidics) [23] , [24] , [25] offers an excellent alternative for the development of tunable, reconfigurable plasmonic devices with multiple functionalities. The optical properties of optofluidic devices can be readily changed by precisely manipulating flow rates and liquid compositions at small spatial scales. In comparison with conventional solid-state devices, the fluidic nature of optofluidic devices enables rapid and dynamic modification of the dielectric environment. As a result, a number of innovative optofluidic technologies have been developed, including optofluidic microscopes [26] , dye lasers [27] , [28] , photonic crystal biosensors [29] , evanescent wave sensor [30] and many others [31] , [32] , [33] , [34] , [35] , [36] , [37] , [38] . Recently, owing to the unique properties of SPPs, researchers have attempted to integrate plasmonics with optofluidics, generating a new branch that has been termed plasmofluidics [39] , [40] , [41] . Bubbles have been previously explored in many microfluidic devices to act as pumps [42] , valves [43] and many others [44] , [45] , [46] . They have also played an important role in modifying properties of plasmonic structures [47] , [48] , [49] , [50] . In this work, we describe a bubble-based plasmofluidic lens that is dynamically tunable and reconfigurable. There are several advantages of using a surface bubble as a plasmonic lens. First, the surface topography, position and shape of a surface bubble, features that collaborate to determine the functionality, can be dynamically controlled and altered. Second, a bubble lens can also be readily erased from the metal surface and replaced by a new lens or lens array. Third, surface bubbles contact the metal film with a contact angle that forms a smooth dielectric interface. This natural dielectric continuously modulates the effective index of SPPs, which may help to reduce scattering loss compared with that of SPP propagation through conventional plasmonic elements fabricated with abrupt discontinuities. In this work, laser-induced surface bubbles on metal films produce the change in the local index for SPPs that propagate along the top surface of the metal. By precisely manipulating the size and location of the surface bubbles, as well as the phase front of the incident SPPs, we have achieved three different functionalities, that is, divergence, collimation, and focusing of SPPs from the plasmofluidic lens. The collimated surface plasmon beam is particularly notable, showing minimal divergence within the measurable 40 μm range. We also show that the shape of the surface bubble can be controlled through a variety of means, considerably expanding the functionality of the plasmofluidic lens. Finally, the refractive index of the liquid solution can be conveniently changed by injecting different liquids and controlling flow rates, offering additional degrees of freedom in the design of plasmofluidic devices. We can also mix fluorescent dye molecules or quantum dots as gain materials into the solution so that the propagation loss of SPPs can be compensated. With these advantages, our findings provide a promising avenue for the design of reconfigurable and multifunctional plasmonic devices for practical applications, and would stimulate continued innovation in the field of plasmofluidics. 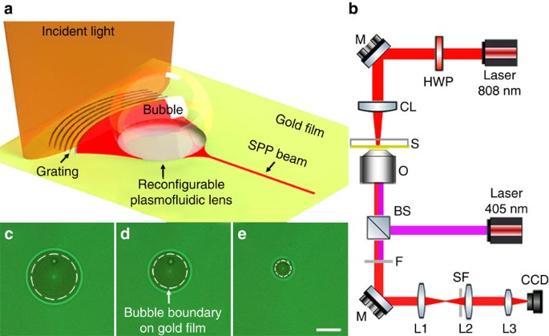Figure 1: Working mechanism of the reconfigurable plasmofluidic lens. (a) Schematic of the reconfigurable plasmofluidic lens, wherein a laser-induced surface bubble is used to control the propagation of SPPs at the metal surface. (b) Schematic of the experimental setup. HWP, half wave plate; M, mirror; CL, cylindrical lens; S, sample; O, oil immersion objective; BS, beam splitter; F, long pass filter; SF, spatial filter; and L, lens. The SPP field is imaged by leakage radiation microscopy, which consists of a high-numerical-aperture oil immersion objective (NA=1.49), three lenses (L1, L2 and L3), and a charge-coupled device camera (CCD). A diode laser with a wavelength of 405 nm is coupled into the leakage radiation microscopy by a beam splitter and focused on the gold surface through the same oil immersion objective. (c–e) Surface bubbles with different diameters (18, 14 and 6 μm, respectively) generated on the gold film. The white dashed circle represents the surface bubble boundary on gold film. Scale bar, 10 μm. Working mechanism of the reconfigurable plasmofluidic lens Figure 1a illustrates the working principle of the reconfigurable plasmofluidic lens. A surface bubble is generated on a metal film by the laser-induced thermal effect in a fluidic environment. As SPPs are sensitive to the index of surrounding materials (solution and vapour in this case), the presence of a surface bubble will strongly alter the propagation of SPPs along the top surface of the metal. In our experimental setup ( Fig. 1b , Methods), a low-power, blue–violet diode laser with a wavelength of 405 nm is employed to generate surface bubbles on a gold film. Here, the gold film has two roles. First, it acts as an effective heat base for bubble generation. Second, it can support SPPs on its surface. The dynamic manipulation of SPPs is achieved by changing the position and size of the surface bubble. When the laser is focused on the gold–water interface, the gold film is quickly heated up, and as a result, a vapour bubble forms around the laser spot on the metal surface. The location and diameter of the vapour bubble can be modulated by moving the laser spot on the gold film and adjusting the laser power, respectively ( Fig. 1c–e ). This kind of flexibility and reconfigurability cannot be easily obtained with a solid-state device. It should be noted that, after its generation, the bubble remains in contact with the gold film, resulting in a truncated sphere shape on the metal film. This allows the SPP field to be greatly modulated by the surface bubble. From the microscope images, we can estimate that the contact angle between the surface bubble and the gold surface is ~ ( Supplementary Fig. S1 ). Figure 1: Working mechanism of the reconfigurable plasmofluidic lens. ( a ) Schematic of the reconfigurable plasmofluidic lens, wherein a laser-induced surface bubble is used to control the propagation of SPPs at the metal surface. ( b ) Schematic of the experimental setup. HWP, half wave plate; M, mirror; CL, cylindrical lens; S, sample; O, oil immersion objective; BS, beam splitter; F, long pass filter; SF, spatial filter; and L, lens. The SPP field is imaged by leakage radiation microscopy, which consists of a high-numerical-aperture oil immersion objective (NA=1.49), three lenses (L1, L2 and L3), and a charge-coupled device camera (CCD). A diode laser with a wavelength of 405 nm is coupled into the leakage radiation microscopy by a beam splitter and focused on the gold surface through the same oil immersion objective. ( c – e ) Surface bubbles with different diameters (18, 14 and 6 μm, respectively) generated on the gold film. The white dashed circle represents the surface bubble boundary on gold film. Scale bar, 10 μm. Full size image Theoretical design guidelines The surface bubble introduces local changes in the effective mode index for SPPs propagating along the gold surface. The effective mode index of SPPs is smaller inside the surface bubble relative to the outside region. 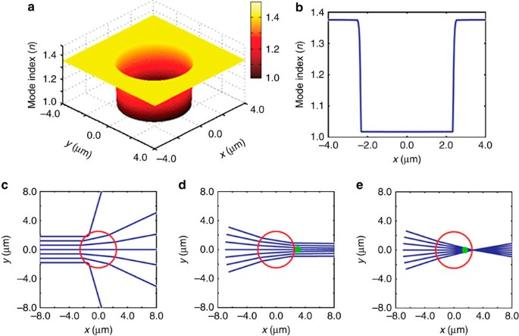Figure 2: Theoretical analysis of the reconfigurable plasmofluidic lens. (a) The distribution of the effective mode index for SPPs at 808 nm wavelength when a surface bubble with a diameter of 5 μm is present on a gold surface. (b) The mode index profile along a straight line across the centre of the bubble. (c–e) Ray tracing results showing SPPs can be diffracted, collimated and focused, respectively, by the plasmofluidic lens. The effective indices inside and outside the bubble are derived from (a). The red circle represents the surface bubble boundary on gold film. The green dot in (d,e) represents the centre of the arc-shaped grating, which is used to excite SPPs with concave phase front. Figure 2a,b shows the effective mode index of SPPs at 808 nm wavelength when a surface bubble with a diameter of 5 μm is present on a gold surface (Methods). It can be seen that the effective mode index quickly reduces from 1.378 (outside the bubble) to 1.020 (inside the bubble). The working principle of the two-dimensional plasmofluidic lens can be best understood through comparison with ray tracing in geometric optics (Methods). As the mode index of SPPs is smaller inside the surface bubble relative to that of the outside, the spherical plasmofluidic lens can be considered as the counterpart of the conventional concave optic lens made of a high-index material (for example, glass) that works in air. If the incident SPPs are plane-wave like (that is, launched from a straight grating with a flat phase front), SPPs refract near the boundaries of the surface bubble and become a diverging beam after passing through the plasmofluidic lens ( Fig. 2c ). This is in direct analogue to the normal glass biconcave or plano-concave lens through which a collimated beam of incident light spreads out in air. To compensate for the spreading, we need to illuminate a focused SPP beam onto the plasmofluidic lens or, equivalently, adjust the phase front of the incident SPPs from flat to concave. Such focused SPPs can be realized with an arc-shaped grating coupler. The resulting characteristics of the SPPs after passing through the lens depend on the curvature of the arc-shaped grating and the diameter and position of the surface bubble. For instance, for a surface bubble with a diameter of 5 μm, SPPs become collimated as shown in Fig. 2d , if the centre of the grating is outside of the surface bubble while being very close to the boundary of the bubble (3.0 μm away from the centre of the bubble). If the curvature of the arc-shaped grating further increases and its centre moves into the surface bubble (1.5 μm away from the centre of the bubble), SPPs are focused near the boundary of the bubble ( Fig. 2e ). Figure 2: Theoretical analysis of the reconfigurable plasmofluidic lens. ( a ) The distribution of the effective mode index for SPPs at 808 nm wavelength when a surface bubble with a diameter of 5 μm is present on a gold surface. ( b ) The mode index profile along a straight line across the centre of the bubble. ( c – e ) Ray tracing results showing SPPs can be diffracted, collimated and focused, respectively, by the plasmofluidic lens. The effective indices inside and outside the bubble are derived from ( a ). The red circle represents the surface bubble boundary on gold film. The green dot in ( d , e ) represents the centre of the arc-shaped grating, which is used to excite SPPs with concave phase front. Full size image Experimental demonstration We start with the experimental demonstration of the divergence of SPPs. 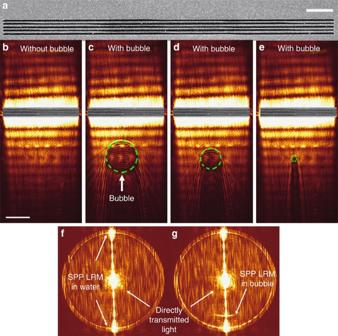Figure 3: Experimental demonstration of SPP divergence by the reconfigurable plasmofluidic lens. (a) Scanning electron microscope image of the fabricated grating. Scale bar, 4 μm. (b) Leakage radiation image of SPPs when surface bubbles are absent. The image was recorded at the image plane. Scale bar, 20 μm. (c–e) Leakage radiation image of SPPs propagating through three surface bubbles with different diameters (27, 17 and 5 μm, respectively). The green dashed circle represents the surface bubble boundary on gold film. (f,g) Fourier plane images of SPPs in the absence and presence of a surface bubble, respectively. Figure 3a shows a scanning electron microscope (SEM) image of the grating used to launch SPPs with a flat wavefront (Methods). After normally illuminating the grating with an 808 nm infrared laser, SPPs with a wavelength of λ spp =585 nm are launched on the gold–water interface. The polarization of the incident light is perpendicular to the grating. The SPP field is imaged using leakage radiation microscopy. Figure 3b is a typical leakage radiation image of SPPs, which shows that SPPs are launched from both sides of the grating. The corresponding image in the Fourier plane is shown in Fig. 3f . The SPP leakage radiation in the Fourier plane is located on a circle as marked by the white arrows. The centre spot in Fig. 3f represents the light that is transmitted directly through the gold film. This light can be blocked by a spatial filter to better articulate the SPP images [51] ( Supplementary Fig. S2 ). The interference pattern that appears in Fig. 3b is a result of coherent superposition of the diffraction-limited imaging of the leakage radiation and SPP coherent propagation [52] . To investigate the effect of the surface bubble on SPP propagation, the laser beam from a blue–violet laser was focused on the gold film and a surface bubble with a diameter of 27 μm was generated 34 μm away from the launching grating. The surface bubble can exist on the gold surface as long as the incident laser keeps heating the gold surface and the entire system maintains the equilibrium state. The surface bubble was observed to maintain its diameter when the laser power was constant ( Supplementary Fig. S3 ). However, when the laser power decreases, the diameter of the surface bubble gradually decreases ( Supplementary Fig. S4 ). Figure 3: Experimental demonstration of SPP divergence by the reconfigurable plasmofluidic lens. ( a ) Scanning electron microscope image of the fabricated grating. Scale bar, 4 μm. ( b ) Leakage radiation image of SPPs when surface bubbles are absent. The image was recorded at the image plane. Scale bar, 20 μm. ( c – e ) Leakage radiation image of SPPs propagating through three surface bubbles with different diameters (27, 17 and 5 μm, respectively). The green dashed circle represents the surface bubble boundary on gold film. ( f , g ) Fourier plane images of SPPs in the absence and presence of a surface bubble, respectively. Full size image Figure 3c–e shows leakage radiation images for SPPs propagating through three surface bubbles with three different diameters (27, 17 and 5 μm, respectively). It is clearly seen that the SPP field is greatly altered by the surface bubble and the SPPs diverge after passing through the lens. Figure 3g shows the image in the Fourier plane after a surface bubble is generated. Compared with Fig. 3f , a new arc appears from SPPs propagating inside the surface bubble, as indicated by the white arrow in Fig. 3g . As the effective mode index of SPPs inside a surface bubble is smaller than that of the surroundings, the leakage radiation image in the Fourier plane of SPPs inside the bubble centres on a circle with a smaller radius than that of outside the bubble. The leakage radiation image recorded in the Fourier plane provides information about the effective mode index of SPPs that propagate on top of the metal film. The effective mode index of the SPPs can be readily obtained from Fig. 3f,g , following the procedure as described by Garcia et al . [53] The centre and outermost edge of the circles in Fig. 3f,g correspond to SPP effective mode indices of 0.0 and 1.49, respectively. The distance from centre and outermost edge of the circle is then used as a scale factor to relate the distance in pixels with a known effective index. The experimental effective mode indices of SPPs in the water and bubble are 1.379 and 1.024, respectively, which agree well with the theoretical values. To compare with the experimental results, finite-difference time-domain (FDTD) simulations are used to calculate the SPP field propagating through a surface bubble (Methods). The results are shown in Supplementary Fig. S5 . One can clearly see that the simulation result agrees with the experimental image very well. In addition to divergence, the plasmofluidic lens enables focusing and collimation of SPPs when the phase front of the incident plasmon waves is concave. 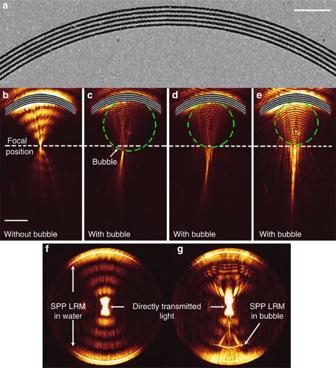Figure 4: Experimental demonstration of SPP focusing and collimation by the reconfigurable plasmofluidic lens. (a) Scanning electron microscope image of the fabricated arc grating. Scale bar, 5 μm. (b) Leakage radiation image of SPPs focused by the arc grating when surface bubbles are absent (the focal position is indicated by a white dashed line). (c–e) Leakage radiation image for SPPs propagating through three surface bubbles with different diameters (45, 39 and 37 μm, respectively). The image was recorded at the image plane. The green dashed circle represents the surface bubble boundary on gold film. Scale bar, 20 μm. (f,g) Fourier plane images of SPPs in the absence and presence of a surface bubble, respectively. Figure 4a shows the SEM image of an arc-shaped grating structure (radius: 38 μm) that was used to generate SPPs with a concave wavefront (Methods). The leakage radiation image for SPPs launched from the curved grating is shown in Fig. 4b . It can be seen that SPPs are focused at the arc’s centre due to constructive interference of SPPs on the focal spot [54] . Here the laser polarization is along the pole of the grating and the focal spot. Figure 4c shows the SPP image when a surface bubble with a diameter of 45 μm is generated between the arc grating and focal spot. In this case, SPPs are tightly focused near the boundary of surface bubble. The diameter of the surface bubble decreases gradually when reducing the blue–violet laser power. Figure 4d,e shows the SPP image when the diameter of the surface bubble was changed to 39 and 37 μm, respectively. As a result, the arc’s centre gradually moves out of the surface bubble. The focal point of SPPs increases, and eventually SPPs become collimated. This trend in SPP propagation agrees with the ray tracing result shown in Fig. 2c–e. Figure 4: Experimental demonstration of SPP focusing and collimation by the reconfigurable plasmofluidic lens. ( a ) Scanning electron microscope image of the fabricated arc grating. Scale bar, 5 μm. ( b ) Leakage radiation image of SPPs focused by the arc grating when surface bubbles are absent (the focal position is indicated by a white dashed line). ( c – e ) Leakage radiation image for SPPs propagating through three surface bubbles with different diameters (45, 39 and 37 μm, respectively). The image was recorded at the image plane. The green dashed circle represents the surface bubble boundary on gold film. Scale bar, 20 μm. ( f , g ) Fourier plane images of SPPs in the absence and presence of a surface bubble, respectively. Full size image Our experimental results indicate that the surface bubble acts as a tunable lens for manipulating SPPs. The focal point can be readily controlled by adjusting the diameter and location of the surface bubble in real time, rendering excellent flexibility for different applications. Figure 4f,g is the leakage radiation images in the Fourier plane before and after the bubble generation, respectively. The angular dependence of the leakage radiation in the Fourier plane reveals the direction of SPP propagation along the gold surface. For a curved grating structure, the propagation direction of SPPs is normal to the curved grating, giving rise to the crescent-shaped pattern in the Fourier plane as shown in Fig. 4f . The two outer light circles marked by the white vertical arrows in Fig. 4f originate from SPPs propagating in opposite directions from both sides of the grating. The leakage radiation image of SPPs inside the bubble is clearly seen in Fig. 4g , located on a circle with a smaller radius. Remarkably, SPPs propagate about 40 μm with minimal divergence when collimated ( Fig. 4e ), in comparison with the decay length of 25 μm for SPPs propagating at the water-gold interface. 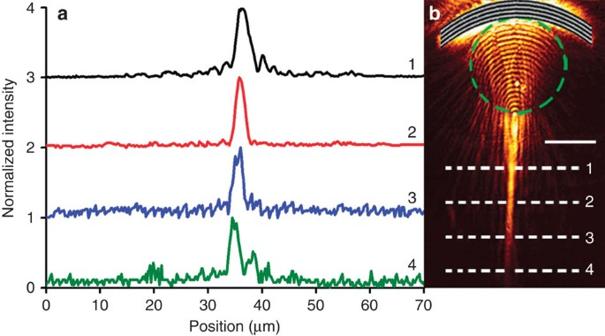Figure 5: SPP intensity distributions along collimated SPP beam. (a) SPP intensity across four different lines (marked by 1, 2, 3 and 4 inb) along its propagation direction. The distance between adjacent lines is 13 μm. The full width at half maximum (FWHM) at four positions (1, 2, 3 and 4) are 2.96, 1.87, 1.95 and 1.84 μm, respectively. (b) Leakage radiation image for collimated SPPs after propagating through a surface bubble with a diameter of 37 μm. The green dashed circle in the inset represents the surface bubble boundary on gold film. Scale bar, 20 μm. Figure 5a presents the SPP intensity distributions across four different lines marked by 1, 2, 3 and 4 (the distance between adjacent lines is 13 μm) along the collimated SPP beam as shown in Fig. 5b . The four curves have been normalized to their maximum intensities. The full width at half maximum of the collimated SPP beam at four positions are 2.96, 1.87, 1.95 and 1.84 μm, respectively, verifying that SPPs propagate a long distance without significant divergence. Our experimental results are further supported by FDTD simulations as shown in Fig. 6 (Methods). 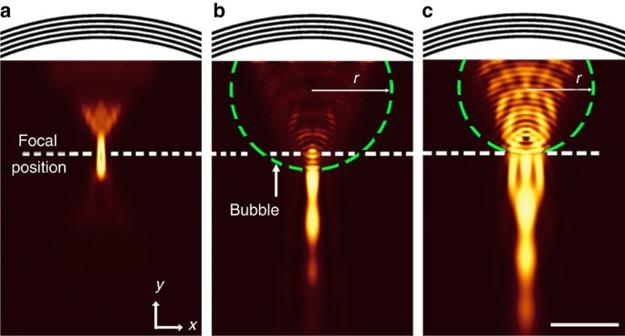Figure 6: FDTD simulation results. (a) SPP field launched by an arc grating without a bubble. (b,c) SPP fields after passing through two surface bubbles with radius of 6 and 5 μm, respectively. The green dashed circle represents the surface bubble boundary on gold film. The white dashed line indicates the SPP focal spot when bubble is absent on the gold film. Scale bar, 5 μm. Figure 6a is the simulation result for the SPP field launched by an arc grating without a bubble, which shows that SPPs are nicely focused at the arc’s centre. Figure 6b,c is the simulation results for SPPs passing through two bubbles of different diameters located between the arc grating and arc centre. The green dashed circles shown in Fig. 6b,c represent the surface bubble boundaries on gold film with radius r =6 and 5 μm, respectively. The white dashed line indicates the SPP focal spot when bubble is absent on the gold surface. From Fig. 6c , one can see that SPPs are well collimated when the front bubble surface is near the focal point of the arc grating, which is in agreement with the experimental results shown in Fig. 4e and 5b . Figure 5: SPP intensity distributions along collimated SPP beam. ( a ) SPP intensity across four different lines (marked by 1, 2, 3 and 4 in b ) along its propagation direction. The distance between adjacent lines is 13 μm. The full width at half maximum (FWHM) at four positions (1, 2, 3 and 4) are 2.96, 1.87, 1.95 and 1.84 μm, respectively. ( b ) Leakage radiation image for collimated SPPs after propagating through a surface bubble with a diameter of 37 μm. The green dashed circle in the inset represents the surface bubble boundary on gold film. Scale bar, 20 μm. Full size image Figure 6: FDTD simulation results. ( a ) SPP field launched by an arc grating without a bubble. ( b , c ) SPP fields after passing through two surface bubbles with radius of 6 and 5 μm, respectively. The green dashed circle represents the surface bubble boundary on gold film. The white dashed line indicates the SPP focal spot when bubble is absent on the gold film. Scale bar, 5 μm. Full size image We have experimentally demonstrated a bubble-based plasmofluidic lens, allowing for the dynamic modulation of SPPs by a surface bubble in a microfluidic environment. The surface bubble was generated by the optothermal effect and remained in tight contact with the gold film on which SPPs were supported. Due to the penetration of the SPPs into the water and surface bubble regions, the effective mode index of the SPPs can be dynamically and spatially modulated as the location and size of the surface bubble changes. The effective index of the SPPs continuously changes on the boundary of the surface bubble due to its naturally smooth contact with the gold film, which may help to reduce the scattering loss relative to SPP propagation through conventional plasmonic elements with abrupt discontinuities. SPP divergence, collimation and focusing were demonstrated using this reconfigurable plasmofluidic lens. The surface bubble can stably exist on the gold film as long as the power of the incident laser maintain constant, as shown in Supplementary Fig. S3 . As a focused laser spot was used to heat the gold film, the generated heat is confined around the laser spot and quickly diffuses through the metal and solution. Therefore, the entire system can operate in a broader temperature range as long as the temperature is below the boiling point and above the freezing point of water. It should be noted that the plasmofluidic lenses are not limited to a spherical shape. A specifically designed shape (such as pentagon, ellipse or parabola shaped bubble) can also be achieved by various means. As shown in Supplementary Figs S6–S9 , we can apply acoustic waves or move laser spot to control the shape of surface bubbles. The functionality of a plasmofluidic lens changes with the shape of the surface bubble as shown in Supplementary Fig. S10 . This provides additional degrees of freedom to enrich the functionality of the plasmofluidic lens. We will continue to explore the performance of these non-spherical plasmofluidic lenses in our future studies. The functionality of our plasmofluidic lens can be further expanded, for example, by introducing fluids with different refractive indices in the microfluidic channel. Optofluidic devices can be tuned by manipulating the refractive index of the liquids, leading us to believe that adjusting the refractive index of the liquids can provide additional tunability and reconfigurability to the plasmofluidic lens presented here. For example, the concentration gradient profile and the corresponding gradient refractive index can be controlled by the flow rate of the core stream and the cladding streams. A complex concentration distribution may allow our device to perform functions beyond plasmofluidic lens, such as plasmofluidic splitting, self-focusing and interference. Finally, it is possible to achieve active plasmonic modulation by injecting liquids mixed with fluorescent dye molecules to act as gain materials in the microfluidic device. One major obstacle hindering the demonstration of plasmonics-based integrated photonic systems is the limited propagation distance of SPPs caused by the intrinsic ohmic loss of metals. This obstacle has stimulated significant interest in exploring the feasibility of achieving SPP loss compensation and lasing by different gain materials, which include fluorescent dye molecules [55] , quantum dots [56] and semiconductors [57] . In our plasmofluidic lens, we are able to mix suitable dye molecules into the solution. Upon optical pumping, the stimulated emission of molecules can amplify the amplitude of SPPs at the probe wavelength. This could lead to plasmonic interconnects or lossless propagation of SPPs, which are required for all-optical devices. In conclusion, our work provides a new paradigm for plasmonics and optofluidics by synergistically combining these two fields. Plasmonics exhibit unique properties of sub-diffraction-limited light confinement and strong local field enhancement, while optofluidics features unparalleled tunability due to the soft, fluidic nature of liquid. Our plasmofluidic lenses pave a new way for designing reconfigurable and multifunctional plasmonic devices in a microfluidic environment. The interplay between plasmonics and optofluidics, such as in the plasmofluidic lens demonstrated here, offers exciting opportunities to advance both fields. It will also likely stimulate new cross-disciplinary technologies for novel applications such as super-resolution imaging, ultra-sensitive biomedical detection and optical information processing. Experimental setup The experimental setup is schematically shown in Fig. 1b . A near infrared diode laser with a wavelength of 808 nm (200 mW) is focused onto a grating by a cylindrical lens to effectively launch SPPs on the gold–water surface. The incident laser polarization is adjusted by a half-wavelength plate. The SPP field is imaged by leakage radiation microscopy, which consists of a high-numerical-aperture oil immersion objective (NA=1.49), three lenses (L1, L2 and L3) and a charge-coupled device camera. By changing the position of the charge-coupled device camera, the Fourier and image plane can be imaged separately and the laser light transmitted directly through the gold film can be blocked with a spatial filter in front of lens 2 (L2). The details of the leakage radiation microscopy can be found in the study of Drezet et al . [51] In order to generate a surface bubble on the gold film, a blue–violet diode laser with a wavelength of 405 nm (100 mW) is coupled with this system by a beam splitter and focused on the gold surface through the same oil immersion objective that is used in the leakage radiation microscopy. The laser power measured before the oil immersion objective is 63 mW. In addition, a long pass filter is placed behind the beam splitter to block light reflected directly from the 405 nm laser. The laser wavelength is chosen to be 405 nm in order to enhance the surface bubble generation; no such effect was observed by using lasers with other wavelengths (for example, 532 or 808 nm) at this power level. Simulation In order to calculate the mode index of SPPs, we use the 2D mode analysis module of the commercial finite-element solver COMSOL 4.3 to solve the SPP wave vector ( β ). The geometry is modelled as layered structures such as water/vapour/gold or water/vapour/water/gold, depending on the position that SPPs reach along the propagating direction. The effective mode index of SPPs is defined as (ref. 58 ). Once the effective mode index distribution is obtained ( Fig. 2a,b ), we can study how SPPs propagate based on a ray tracing technique [59] ( Fig. 2c–e ). We perform full-wave FDTD simulations (lumerical) to model the behaviour of the reconfigurable plasmonic lens. Instead of simulating the real geometry used in the experiment, a straight grating with a reduced width and length of 2.6 and 20 μm is used to conduct the simulation in Supplementary Fig. S5b to save computation resources. The surface bubble with radius r =5 μm on gold film is 4.5 μm away from the grating. An arc grating with a reduced length and radius of 13 and 10 μm is used in the simulation in Fig. 6 . Sample fabrication A 50 nm Au film was evaporated onto a cover glass. The grating used to launch SPPs was fabricated on the gold film by a focused-ion beam machine (Quanta 200 3D, FEI). The straight grating that was used to launch SPPs with flat wavefront has a slit-to-pitch ratio of 0.5 and period λ spp =585 nm, where λ spp is the wavelength of SPPs as shown in Fig. 3a . The slit width was 292 nm and the total width and length of the grating were 2.6 and 60 μm, respectively. The arc grating structure that was used to launch SPPs with concave wavefront consists of five concentric slits as shown in Fig. 4a . The width and period of the slits are chosen to be 292 and 585 nm, respectively, in order to effectively launch SPPs on the gold–water interface. The length and radius of the arc grating are 60 and 38 μm, respectively. A microfluidic chamber containing water with a depth of 170 μm is then added on top of the gold film. How to cite this article: Zhao C. et al . A reconfigurable plasmofluidic lens. Nat. Commun. 4:2305 doi: 10.1038/ncomms3305 (2013)